Discovery of LaAlO3as an efficient catalyst for two-electron water electrolysis towards hydrogen peroxide Electrochemical two-electron water oxidation reaction (2e-WOR) has drawn significant attention as a promising process to achieve the continuous on-site production of hydrogen peroxide (H 2 O 2 ). However, compared to the cathodic H 2 O 2 generation, the anodic 2e-WOR is more challenging to establish catalysts due to the severe oxidizing environment. In this study, we combine density functional theory (DFT) calculations with experiments to discover a stable and efficient perovskite catalyst for the anodic 2e-WOR. Our theoretical screening efforts identify LaAlO 3 perovskite as a stable, active, and selective candidate for catalyzing 2e-WOR. Our experimental results verify that LaAlO 3 achieves an overpotential of 510 mV at 10 mA cm −2 in 4 M K 2 CO 3 /KHCO 3 , lower than those of many reported metal oxide catalysts. In addition, LaAlO 3 maintains a stable H 2 O 2 Faradaic efficiency with only a 3% decrease after 3 h at 2.7 V vs. RHE. This computation-experiment synergistic approach introduces another effective direction to discover promising catalysts for the harsh anodic 2e-WOR towards H 2 O 2 . Hydrogen peroxide (H 2 O 2 ) is an environmentally benign and powerful chemical oxidizer widely used in electronics manufacturing [1] , [2] , chemical synthesis [3] , [4] , water purification [5] , and many other industrial sectors. Currently, H 2 O 2 is produced by the anthraquinone process, which necessitates an energy-demanding multi-electron process and massive infrastructures to transport it to the point of use [6] . Recently, electrochemical processes, such as two-electron oxygen reduction reaction (2e-ORR) and water oxidation reaction (2e-WOR) [7] , [8] , [9] , have emerged as attractive routes to produce H 2 O 2 onsite in small-scale distributed units [10] . The 2e-ORR has been extensively investigated, and many suitable catalysts with high activity and selectivity have been reported, including noble metals [10] , [11] , [12] , carbon materials [13] , [14] , and transition metals [15] , [16] . Unlike 2e-ORR which needs oxygen, the 2e-WOR only requires water as a reactant, thus simplifying the system for the synthesis of H 2 O 2 . The pioneering research on H 2 O 2 production via 2e-WOR in 2004 showed the feasibility of this process using a carbon-based catalyst in the alkaline electrolyte [17] . Most recent reports on the 2e-WOR catalysts have focused on using metal oxides [18] , [19] , [20] , [21] , [22] , [23] , [24] , doped metal oxides [25] , [26] , heterostructure [27] , [28] , carbon-based materials [29] , [30] , [31] , and electrolyte engineering [32] , [33] . However, the 2e-WOR still needs significant improvement in electrocatalysts to be more stable, active, and selective. The elementary steps for the 2e-WOR are associated with the interaction between the catalyst surface and oxygen intermediates: *O, *OH, and *OOH [34] . For a catalyst to be selective for the 2e-WOR, the binding energy of those intermediates should be in the right range. If the binding is too strong, the adsorbed OH* is further oxidized to *O and *OOH, facilitating 4e-WOR for O 2 evolution. If the binding is too weak, it is difficult to activate the water molecule and form the *OH. Currently, for 2e-WOR, the state-of-the-art metal oxide catalysts still show more than 1 V overpotential from the equilibrium potential for H 2 O 2 (1.76 V vs. RHE) to reach 10 mA cm −2 of the current density [18] , [19] , [21] , [25] . Recently, perovskite oxides have garnered significant attention in numerous applications, such as electronics [35] , energy conversion and storage [36] , and catalysts [37] , [38] . Perovskites have a unit formula ABO 3 , where A cation sites are usually rare-earth or alkaline earth metal, and B cations are typically small transition metal elements staying at the centre of the oxygen octahedron [39] . Perovskites incorporate a broad combination of A and B cations, using more than 90% of metallic elements in the periodic table [39] . As such, perovskites provide rich opportunities to tune their chemical, physical, and catalytic properties. A superior catalyst for 2e-WOR must meet the following three requirements: (i) high stability to fulfil the demand for long-term operation; (ii) high selectivity to prevent the formation of by-products; (iii) high activity to save energy input. We investigated the stability through a computational screening of a vast number of perovskites in the Materials Project database [40] as suggested by Persson et al. [41] This approach has proven to be powerful in rapidly excluding a variety of catalyst materials that do not fall within the desired stability target for long term and practical application. This approach was first introduced by Persson et al. to discover synthesizable and robust photocatalysts for CO 2 reduction reactions via computational analysis [42] . The recent work by Gunasooriya and Nørskov is another example of applying this approach to discovering stable oxides for the oxygen reduction reaction [43] . Following this approach, we study an extensive library of more than 2000 perovskites to identify 32 stable perovskites at pH = 8 and 10 stable perovskites at pH = 11, conditions relevant for 2e-WOR. Among the 32 stable perovskites, LaAlO 3 stands out as the most stable perovskite from this study. We further study the activity and selectivity of a series of four other Lanthanum-based (La-based) perovskites including LaCuO 3 , LaNiO 3 LaGaO 3 , and LaZnO 3 using density functional theory (DFT) calculation and reported data in the literature [44] , [45] . We show that LaAlO 3 is not only the most stable but also the most active and selective catalyst for 2e-WOR among other stable La-based perovskites. It is also the most active, selective, and stable material reported so far [8] , [18] , [19] , [21] , [25] , [46] . To verify the computational prediction, we synthesize LaAlO 3 thin films on FTO glass using the solution-combustion method. The synthesized LaAlO 3 thin film is confirmed to have a cubic perovskite crystal structure with the dominant phases of (110) and (111) through transmission electron microscopy (TEM), grazing-incidence X-ray diffraction (GIXRD), and X-ray photoelectron spectroscopy (XPS) analysis. Moreover, the LaAlO 3 thin film has excellent catalytic properties towards 2e-WOR, with an onset potential of 510 mV at 10 mA cm −2 , a peak faradaic efficiency (FE) of 87% at 3.34 V vs. RHE, H 2 O 2 production rates of 0.16 mmol cm −2 (128 ppm) and 1.23 mmol cm −2 (808 ppm) at 2.7 and 3.2 V vs. RHE after 3 h, and good stability over 3 h of testing, supporting the theoretical results. Computational analysis As discussed above, stability is a major challenge for catalysts under the harsh anodic oxidation potential conditions required for 2e-WOR toward H 2 O 2 production. Under highly oxidizing 2e-WOR conditions, lack of catalyst stability is a major cause of catalyst degradation, resulting in a loss of catalytic activity and selectivity [25] . Thus, we first place a particular emphasis on filtering the stable perovskites out of more than 2,000 ABO 3 structures (Fig. 1 ). We applied three stability criteria. First, the decomposition energy, defined as a difference between the Gibbs free energies of perovskites and the most stable product they are decomposed to in aqueous media [41] , to be <0.1 eV. The selection of the 0.1 eV threshold was based on the recommendation by Persson et al. to assure the highest stability for perovskites [47] . The second criterion is to be stable under electrochemical conditions (pH = 8 and pH = 11 with applied electrode potentials of 2.23 and 2.41 V versus SHE, respectively) using Pourbaix diagram analyzer using Python Material Genome (Pymatgen) [48] and Materials Project [40] cooperatively. The pH=8 and pH=11 were chosen because they are the operating conditions in most experimental studies for 2e-WOR [18] , [29] . The last criterion is only to include structures with cubic \({Pm}\bar{3}m\) space group and a larger A cation as they are the most stable and typical crystal structures for ABO 3 perovskites. The use of these three criteria yields 10 (Fig. 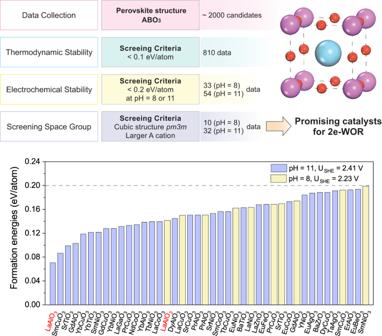Fig. 1: Computational screening to discover the most stable perovskite oxide under different pH conditions. Filtering stable ABO3perovskite structures based on three screening criteria including decomposition energy < 0.1 eV and electrochemical stability under pH = 8 and 11. 1 and Supplementary Table 1 ) and 32 (Fig. 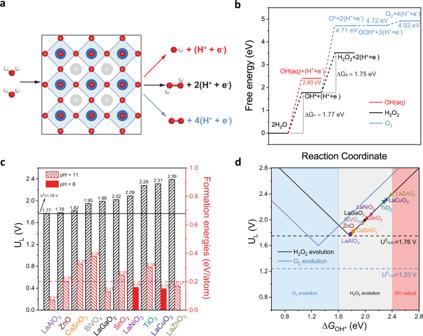Fig. 2: Mechanism of the 2e-WOR H2O2production in LaAlO3and comparison of limiting potential and formation energy with different catalysts. aWOR processes via different pathways. La, Al, O, and H are represented by gray, blue, red, and white spheres, respectively.bFree energy diagram of all the three WORs over LaAlO3.cCalculated limiting potentials (UL, left axis) for the metal oxides, and the corresponding formation energies (right axis) under 2e-WOR (electrolyte pH = 11 or 8).dVolcano plots of limiting potential as a function of ΔGOH*. 1 and Supplementary Table 2 ) stable perovskites at pH = 8 and 11, respectively. Among them, LaAlO 3 was identified as the most stable with the least formation energy at both pH values (pH = 8 and 11). Additionally, the superior stability of LaAlO 3 has been revealed by the extremely high O-vacancy formation energy of 2.91 eV, as shown in Supplementary Fig. 1 . The less stable perovskites with higher formation energies are more likely to suffer from catalyst aging, thereby resulting in catalyst deactivation and the demand of more frequent catalyst replacement in the device to maintain a target level of H 2 O 2 production. We note that the stability analysis based on the Pourbaix diagram analyzer, introduced by Persson et al. [41] is established based on sole thermodynamic analysis with no consideration of the possible kinetic stability as a result of the slow dissolution process or formation of resistant films on the catalyst surface under reaction conditions. Previous studies show that materials such as BiVO 4 [25] for the 2e-water oxidation reaction that does not come out as a stable material from the Pourbaix diagram analysis can survive the anodic reaction conditions for several hours. On the other hand, approaches can be taken to increase the stability of those materials. For example, doping BiVO 4 with Gadolinium has been used as a strategy to improve the long-term stability of BiVO 4 by preventing the leaching of vanadate ions [25] . In this work, we used the Pourbaix Diagram analysis to mark the materials that inherently have high stability, not taking into account the ones that may not be thermodynamically stable but may show kinetic stability as a result of a slow dissolution process under reaction conditions or those that may make a resistant film under reaction conditions. Moreover, since LaAlO 3 is the most stable perovskite under 2e-WOR conditions, it is highly promising to eliminate the effect of catalyst degradation, maintain catalytic performance and extend its stability to meet the long-term operation targets. Apart from the exceptional stability, LaAlO 3 is earth-abundant and non-toxic, providing a potential to investigate the 2e-WOR activity for LaAlO 3 , which will be described in the later section. Fig. 1: Computational screening to discover the most stable perovskite oxide under different pH conditions. Filtering stable ABO 3 perovskite structures based on three screening criteria including decomposition energy < 0.1 eV and electrochemical stability under pH = 8 and 11. Full size image Next, we employed DFT calculation to evaluate the theoretical activity and selectivity of LaAlO 3 for 2e-WOR. Water oxidation may follow four-electron, two-electron, and one-electron pathways (Fig. 2a ); hence selectivity toward H 2 O 2 product is a great challenge. Previous studies have identified that the binding energies of different reaction intermediates (O*, OH*, and OOH*) are suitable descriptors for the activity and selectivity of water oxidation reaction pathways [7] , [8] . An active catalyst for 2e-WOR has an optimum OH* binding (Δ G OH* ≥ 1.76 eV with reference to H 2 O). In order to be selective, the catalyst should weakly bind O* (Δ G O* ≥ 3.52 eV) to suppress the 4e-WOR route and prevent the further oxidation of H 2 O 2 to O 2 . Moreover, the catalyst should bind OH* below 2.4 eV (Δ G OH* < 2.4 eV) to avoid the formation and release of OH radicals. For LaAlO 3 (100) surface, the adsorption energies of these critical intermediates are Δ G OH* = 1.77 eV and Δ G O* = 4.71 eV (Supplementary Fig. 2 ). Thus, LaAlO 3 is highly selective and active for the 2e-WOR and suppresses both the 1e- and the 4e-WOR pathways, as shown in Fig. 2b . Note that the (100) facet of LaAlO 3 was used in this analysis, as it is predicted as the most stable among (100), (110), and (111) facets based on surface energy calculations (Supplementary Fig. 3 ). Fig. 2: Mechanism of the 2e-WOR H 2 O 2 production in LaAlO 3 and comparison of limiting potential and formation energy with different catalysts. a WOR processes via different pathways. La, Al, O, and H are represented by gray, blue, red, and white spheres, respectively. b Free energy diagram of all the three WORs over LaAlO 3 . c Calculated limiting potentials (U L , left axis) for the metal oxides, and the corresponding formation energies (right axis) under 2e-WOR (electrolyte pH = 11 or 8). d Volcano plots of limiting potential as a function of Δ G OH* . Full size image In addition to LaAlO 3 , we investigated the 2e-WOR of four other La-based perovskites that were identified as stable materials in Fig. 1 . We performed explicit calculations for LaCuO 3 and LaNiO 3 (Supplementary Fig. 4 ) and data for LaGaO 3 and LaZnO 3 were extracted from the literatures [44] , [45] . The calculated limiting potential (U L ) and relative stability of LaAlO 3 are compared in Fig. 2c to four other La-based perovskites as well as several oxides that have been evaluated for 2e-WOR [18] , [19] . The solid upper line marks the thermodynamic potential of 1.76 V for 2e-WOR. The lower dashed line indicates the electrochemical stability with a formation energy of 0.2 eV/atom. Figure 2c shows that LaAlO 3 is the most active La-based perovskite (with the lowest calculated limiting the potential of 1.77 eV) and the most stable (pH = 11, results for pH = 8 in Supplementary Fig. 5 ) catalyst among previously reported oxides under 2e-WOR conditions. Figure 2d shows the U L vs. Δ G OH* for those oxides and perovskites. The binding of OH* on the LaAlO 3 surface is 1.77 eV which is the closest to the optimal value of 1.76 eV. In addition, we performed the Bader charge analysis to understand the active site in LaAlO 3 (Supplementary Fig. 6 ). Our results revealed a strong electron-accepting feature on the Al sites, characterized by higher charges (+2.41 to +2.43 e) as compared to the ones on La (+2.05 to +2.07 e) coming from its oxophilic nature. These more positive charges can facilitate the adsorption of negatively charged OH species in the alkaline electrolyte and thereby increase the activity of LaAlO 3 toward 2e-WOR. To understand the contribution of O-vacancies and defects in the activity of LaAlO 3 , we calculated the OH* adsorption on LaAlO 3 with O-vacancy (Supplementary Fig. 1c ). The O-vacancies are strongly binding to the OH* intermediate (Δ G OH* = −2.51 eV), indicating the O-vacancies do not contribute to the 2e-WOR. Since the formation of additional O-vacancies in LaAlO 3 is strongly endothermic (by ~3 eV) as stated above, it is unlikely for LaAlO 3 to form additional defects under 2e-WOR conditions. Thus, according to the DFT results, LaAlO 3 is the stable, active, and selective catalyst for 2e-WOR. We note that the carbonate anion has also been considered in the H 2 O 2 reaction calculation since it is essential in the commonly used electrolyte (2 M KHCO 3 ) [18] , [32] , [49] . To evaluate the effect of carbonate anion on H 2 O 2 production, we calculated the 2e-WOR pathway with carbonate anion as a mediator as reported by Fan et al. (Supplementary Fig. 7 ) [50] . This analysis shows that the largest free energy change via carbonate mediated pathway is 2.03 eV to generate H 2 O 2 , indicating that the theoretical limiting potential is 2.03 V, slightly higher than that of 2e-WOR pathway without carbonate (1.77 V). Additionally, we calculated the H 2 CO 3 oxidation mechanism proposed by Kusama et al. (Supplementary Fig. 8 ) on the LaAlO 3 surface [51] . Our results agree well with the report by them and show that the first proton removal from the adsorbed H 2 CO 3 is the rate-limiting step. The energy difference we calculated for this step is 1.89 eV, indicating a limiting potential of 1.89 V. This limiting potential of 1.89 V is also slightly (~0.1 V) higher than the value calculated for 2e-WOR on bare LaAlO 3 (1.77 V). However, all these three values (2.03, 1.77 and 1.89 V) are reasonably close, and under the operating reaction potentials all pathways will be accessible. Thus, we conclude that the carbonate and H 2 CO 3 oxidation provide additional pathways to promote the H 2 O 2 production. Synthesis of LaAlO 3 perovskite oxide catalyst The synthesis of LaAlO 3 perovskite oxide requires a high temperature of 800–1700 ˚C to obtain a pure cubic crystal structure with a space group of \({Pm}\bar{3}m\) , and LaAlO 3 has been synthesized by methods such as the solid-state reaction of Al 2 O 3 and La 2 O 3 [52] , [53] , co-precipitation [54] , aerosol technique [55] , and sol-gel method [56] , [57] . To remove the need for such a high-temperature source, we employed a self-sustaining solution-based combustion synthesis method [58] , [59] to prepare LaAlO 3 that requires heating only at 300 ˚C. As illustrated in Fig. 3a , acetylacetone (C 5 H 8 O 2 ) and metal nitrates serve as fuel and oxidizers, and their reaction onset temperature is about 240 ˚C as determined by the thermogravimetric analysis (TGA) and differential scanning calorimeter (DSC) measurement (Supplementary Fig. 9 ). The mixture of metal nitrates and acetylacetone was spin-coated on an FTO glass, and we set the hot plate at 300 °C to have sufficient temperature to initiate their exothermic reaction, and the generated heat enabled the conversion of the metal precursors to LaAlO 3 and other gaseous products. The synthesis conditions, in terms of the precursor ratio, processing temperature, and the number of coating layers on the activity, are summarized in Supplementary Fig. 10 . Fig. 3b shows the top-view scanning electron microscopy (SEM) image of as-synthesized LaAlO 3 on the FTO glass. The bare FTO has grains of several hundred nanometers scale with smooth surfaces. After the LaAlO 3 film is deposited on top, the FTO glass looks similar, but the grain surface looks rougher and more wrinkled, which looks like 2D sheets with a thickness of roughly 20–30 nm (Supplementary Fig. 11 ). The transmission electron microscopy (TEM) dark-field image and energy-dispersive X-ray spectroscopy (EDS) elemental analysis in Fig. 3c and SEM-EDS mapping images on several spots throughout the film in Supplementary Fig. 11 show that all elements (La, Al, and O) are uniformly distributed throughout the whole area of the film. Fig. 3: Solution combustion synthesis process and characterizations of the final product. a Schematic of low-temperature solution combustion processing mechanism for LaAlO 3 synthesis. b SEM top-view and c TEM dark-field and EDS mapping images of the synthesized LaAlO 3 . Full size image Material characterizations of LaAlO 3 perovskite High-resolution TEM (HRTEM) images of LaAlO 3 in Fig. 4a reveal that the particles are composed of both amorphous and crystalline parts (yellow circles). As shown in Fig. 4b, c , and Supplementary Fig. 12 , HRTEM images show that the cubic structure with a space group of \({Pm}\bar{3}m\) of the LaAlO 3 phase belongs to the (100) and (110) planes, which has a lattice spacing of 3.8 and 2.7 Å, respectively. Moreover, these planes in \({Pm}\bar{3}m\) space group have formation energies of 0.11 and 0.28 eV/atom, which is favorable for 2e-WOR from the DFT calculations in Supplementary Fig. 3 . In addition to the TEM analysis, the Grazing-incidence X-ray diffraction (GIXRD) measurement in Fig. 4d shows that the formed crystalline particles on FTO have the LaAlO 3 perovskite structure (ICDD 01–083–4238), for which the peak at 11.46 ° corresponds to the (100) plane. The 15.7° peak is overlapped by the (110) peak of LaAlO 3 and the FTO substrate peak; however, the HRTEM confirms the (110) facet for LaAlO 3 . Since the GIXRD was collected with the X-rays with its incident energy of 17.0 keV and wavelength of 0.729 Å [60] , the two theta values are different from those with the general Cu Kα (1.54 Å). All the above results confirm that the crystal structure of LaAlO 3 is cubic perovskite. Fig. 4: Key characterizations of the synthesized LaAlO 3 . a – c High-resolution TEM images of LaAlO 3 synthesized by sol-gel combustion method. From the TEM images, the morphology shows an irregular shape with the size of several tens of nm. And most of the parts look amorphous, while a crystalline LaAlO 3 phase was created at some surface parts. This resulted from the temperature spontaneously attained during the combustion process instantaneously that extends to the range of 2000 °C for short periods. d GIXRD result of LaAlO 3 on FTO/glass substrate, e Surface analysis using XPS survey spectra with the inlet table with the elemental concentration (%), and the detailed elemental regions: f La 3d, g Al 2p, and h O 1 s. Full size image In addition, X-ray photoelectron spectroscopy (XPS) was performed to investigate the surface elemental components of the as-synthesized LaAlO 3 . The XPS survey profile in Fig. 4e shows that the elemental ratio between La and Al was approximately 1. The high-resolution XPS spectra in Fig. 4f show that the La 3d core level splits into 3d 3/2 and 3d 5/2 components due to the spin-orbit coupling. The observed La 3d 5/2 doublet has a splitting of ~4.0 eV, which agrees with the formation of lanthanum oxide [61] , [62] . In comparison, the sol-gel synthesized LaAlO 3 has a La 3d 5/2 doublet of about 3.7 eV, which indicates lanthanum hydroxide species (Supplementary Fig. 13 ). Furthermore, the O 1 s core level for combustion-synthesized LaAlO 3 in Fig. 4h consists of three peaks: La–O, La–O–Al, and Al–O at 529 eV, 530.1 eV, and 531.2 eV, respectively [63] , [64] , [65] . In another way, the deconvoluted O 1s peak also contains a slight amount of oxygen vacancies in the lattice and the ratio between the oxide and oxygen vacancy is approximately 10:1 based on their integrated areas, which can contribute to the conductivity of LaAlO 3 (Supplementary Fig. 14 ). The O 1 s peaks for sol-gel synthesized LaAlO 3 imply that the surface contains the hydroxide species rather than the oxides (Supplementary Fig. 13 ). Those analyses indicate that the solution-based combustion reaction effectively converts the metal precursors into crystalline perovskite oxide [58] , [66] . Evaluation of electrocatalytic H 2 O 2 evolution properties on LaAlO 3 perovskite oxide Figure 5a plots the linear sweep voltammetry (LSV) curves of the combustion-synthesized LaAlO 3 on FTO/glass and the bare FTO/glass in two different electrolytes: 2 M KHCO 3 (pH = 8.3) and 4 M K 2 CO 3 /KHCO 3 (molar ration of 1:7, pH = 11). The 2 M KHCO 3 is the commonly used electrolyte for 2e-WOR [18] , [32] , [49] , while the 4 M K 2 CO 3 /KHCO 3 electrolyte was recently identified as a better electrolyte with higher selectivity towards 2e-WOR [33] , [67] . 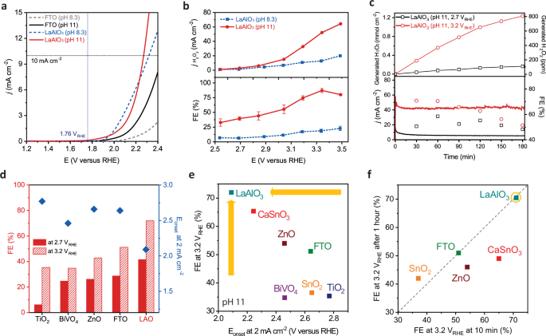Fig. 5: Electrochemical performance. aLinear sweep voltammetry curves of LaAlO3anode compared to FTO/glass substrate in the electrolyte of 2 M KHCO3(pH 8.3) and 4 M K2CO3/KHCO3(pH 11). All curves are 95 % iR-compensated.bThe calculated H2O2current density and selectivity of LaAlO3anode as a function of potential in different electrolytes, andcthe generated H2O2amount, selectivity, and stability of the LaAlO3anode at different potentials, 2.7 and 3.2 V vs. RHE for 3 h.dComparison of Faradaic efficiencies at different potentials and onset potentials to reach 2 mA cm−2with the previously reported materials in pH 11.eSelectivity vs. activity plot for different metal oxides in the electrolyte of 4 M K2CO3/KHCO3(pH 11) at 3.2 V vs. RHE.fComprehensive plot for selectivity and stability in the electrolyte of 4 M K2CO3/KHCO3(pH 11) at 3.2 V vs. RHE. Thex-axis is the FE at timet= 10 min. They-axis is the FE at timet= 1 h. The diagonal dashed line is the expected response for a stable catalyst. Indeed, both LaAlO 3 /FTO and bare FTO exhibit earlier onset potentials in the newly optimized 4 M K 2 CO 3 /KHCO 3 electrolyte. The overpotentials at 10 mA cm −2 of LaAlO 3 /FTO film were measured to be 560 mV in 2 M KHCO 3 and 510 mV in 4 M K 2 CO 3 /KHCO 3 (equilibrium potential: 1.76 V vs. RHE). In both electrolytes, the overpotentials of LaAlO 3 /FTO are smaller than those of bare FTO. The electrochemical impedance spectroscopy (EIS) analysis was conducted to compare the conductivity of LaAlO 3 and FTO substrate at 2.7 V vs. RHE (Supplementary Fig. 15 ). The data were fitted with a REAP2CPE equivalent circuit model in which there were three types of resistances: resistance in the electrolyte solution (R1), charge transfer resistance inside bulk catalyst (R2), and charge transfer resistance at the interface between the catalyst and electrolyte (R3). Here, we could emphasize R2 and R3 values, which contribute to the conductivity inside the bulk of the catalyst material and at the interface between the material surface and the electrolyte. Here, LaAlO 3 film shows roughly 3.5 times lower bulk and interface resistances than FTO itself at 2.7 V vs. RHE, which is the desired potential for H 2 O 2 production. This presumably results from the oxygen vacancy in the lattice (Supplementary Fig. 14 ). This can also be evidence that our LaAlO 3 is not an insulating material compared to FTO. In addition, we also measured the activity for some stable perovskite oxides, based on the formation energies (Fig. 1 ), in 4 M K 2 CO 3 /KHCO 3 (pH 11; Supplementary Fig. 16 ). All perovskite oxides here were synthesized by the same method as that for LaAlO 3 . We found that SmCuO 3 and GdCuO 3 also showed relatively good activity (610 and 660 mV at 10 mA cm −2 , respectively) but were still inferior to the activity of LaAlO 3 . Figure 5b shows that the H 2 O 2 current densities (j H2O2 ) and the Faradaic efficiencies (FE) of LaAlO 3 /FTO are higher in 4 M K 2 CO 3 /KHCO 3 (pH 11) than those in 2 M KHCO 3 (pH 8.3), especially at higher bias, and the peak FE reaches 87 % at 3.34 V vs. RHE in the optimized electrolyte vs. 23 % at 3.5 V vs. RHE in 2 M KHCO 3 (see Methods section for details). We further tested the stability of LaAlO 3 /FTO in 4 M K 2 CO 3 /KHCO 3 under two current densities of 3 and 33 mA cm −2 at 2.7 and 3.2 V vs. RHE, respectively. Figure 5c shows that the LaAlO 3 /FTO has a smaller FE decrease at 2.8 V vs. RHE (from 51% to 48%) than at 3.2 V vs. RHE (70% to 51%) after 3 h of the test. After 3 h of the durability test, 0.16 mmol cm −2 (128 ppm) and 1.23 mmol cm −2 (808 ppm) of H 2 O 2 were generated at 2.7 and 3.2 V vs. RHE, respectively, in comparison to only 70 μmol cm −2 at 2.7 V vs. RHE for bare FTO (Supplementary Fig. 17 ). After the stability test, we measured the post-situ XPS and SEM images to assess any elemental composition and morphology changes (Supplementary Figs. 18 and 19 ). No compositional degradations in La 3d , Al 2p , and O 1 s regions were observed from the post-situ XPS analysis after 3 h of the durability test nor any morphological degradation from the SEM images. Fig. 5: Electrochemical performance. a Linear sweep voltammetry curves of LaAlO 3 anode compared to FTO/glass substrate in the electrolyte of 2 M KHCO 3 (pH 8.3) and 4 M K 2 CO 3 /KHCO 3 (pH 11). All curves are 95 % iR-compensated. b The calculated H 2 O 2 current density and selectivity of LaAlO 3 anode as a function of potential in different electrolytes, and c the generated H 2 O 2 amount, selectivity, and stability of the LaAlO 3 anode at different potentials, 2.7 and 3.2 V vs. RHE for 3 h. d Comparison of Faradaic efficiencies at different potentials and onset potentials to reach 2 mA cm −2 with the previously reported materials in pH 11. e Selectivity vs. activity plot for different metal oxides in the electrolyte of 4 M K 2 CO 3 /KHCO 3 (pH 11) at 3.2 V vs. RHE. f Comprehensive plot for selectivity and stability in the electrolyte of 4 M K 2 CO 3 /KHCO 3 (pH 11) at 3.2 V vs. RHE. The x -axis is the FE at time t = 10 min. The y -axis is the FE at time t = 1 h. The diagonal dashed line is the expected response for a stable catalyst. Full size image Figure 5d compares the FEs (right) at 2.7 and 3.2 V vs. RHE of LaAlO 3 /FTO and the onset potential to attain 2 mA cm −2 (left) with previously reported metal oxide catalysts on FTO in the same electrolyte (4 M K 2 CO 3 /KHCO 3 ). The LaAlO 3 perovskite oxide exhibits much higher FEs and lower onset potential than TiO 2 , BiVO 4 , ZnO, and FTO. Additionally, LaAlO 3 has the lowest overpotential to reach 2 mA cm −2 among all the previously reported metal oxides in 2 M KHCO 3 in Supplementary Fig. 20. Furthermore, we conducted the activity, stability, and selectivity test for some of the state-of-the-art metal oxides (CaSnO 3 , ZnO, and SnO 2 ) to compare with those for LaAlO 3 in 4 M K 2 CO 3 /KHCO 3 (pH 11), showing that LaAlO 3 exhibited the lower overpotential, higher FEs and generated H 2 O 2 amount (Supplementary Fig. 21 ). Other oxides (BiVO 4 , TiO 2 , ZnO, and FTO) were investigated for electrochemical H 2 O 2 production under the same condition in our previous study [32] , [67] . In Supplementary Fig. 22 (Reprinted (adapted) with permission from ref. 68 . Copyright 2021 American Chemical Society.) [68] , the production rate of H 2 O 2 for LaAlO 3 is much higher than other reported metal oxides and similar to the boron-doped diamond (BDD). Finally, we assessed different state-of-the-art metal oxides by plotting FEs at 3.2 V RHE vs. onset potential to reach 2 mA cm −2 in 4 M K 2 CO 3 /KHCO 3 (pH 11) in Fig. 5e . LaAlO 3 is positioned at the very upper left side of the plot, which means the most active and selective catalyst among different metal oxides. Figure 5f also demonstrates the comprehensive plot for the selectivity and stability in 4 M K 2 CO 3 /KHCO 3 (pH 11) at 3.2 V vs. RHE. 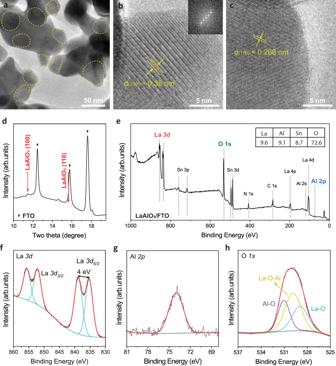The x -axis is the FE at t = 10 min, and the y -axis is the FE at t = 1 h. The diagonal dashed line is the expected response for a stable catalyst. Fig. 4: Key characterizations of the synthesized LaAlO3. a–cHigh-resolution TEM images of LaAlO3synthesized by sol-gel combustion method. From the TEM images, the morphology shows an irregular shape with the size of several tens of nm. And most of the parts look amorphous, while a crystalline LaAlO3phase was created at some surface parts. This resulted from the temperature spontaneously attained during the combustion process instantaneously that extends to the range of 2000 °C for short periods.dGIXRD result of LaAlO3on FTO/glass substrate,eSurface analysis using XPS survey spectra with the inlet table with the elemental concentration (%), and the detailed elemental regions:fLa 3d,gAl 2p, andhO 1 s. LaAlO 3 is located on both the expected response line and the highest FE region, which indicates the most selective and stable catalyst among the known state-of-the-art metal oxides. These results indicate that the LaAlO 3 catalyst has superior activity and selectivity for 2e-WOR to produce H 2 O 2 , especially in the recently optimized 4 M K 2 CO 3 /KHCO 3 electrolyte. Here, we utilized combined computational screening and experimental results to identify LaAlO 3 as the most stable, active, and selective catalyst reported thus far for 2e-WOR to H 2 O 2 production. First, we extensively investigated a library of more than 2000 perovskites to identify 32 stable perovskites at pH=8 and 10 stable perovskites at pH = 11 for 2e-WOR. Among them, LaAlO 3 was found as the most stable with the smallest formation energy under both pH conditions. Then, in order to provide a potential to examine the 2e-WOR activity, we synthesized LaAlO 3 via self-sustaining solution-combustion method. The synthesized LaAlO 3 exhibits a cubic crystal structure with dominant planes of (100) and (110). The catalytic properties of LaAlO 3 towards 2e-WOR were evaluated at two different electrolytes: 2 M KHCO 3 (pH 8.3) and 4 M K 2 CO 3 /KHCO 3 (1:7, pH 11), and LaAlO 3 shows better activity towards 2e-WOR than TiO 2 , BiVO 4 , ZnO, and FTO in both electrolytes. LaAlO 3 achieves a superior 2e-WOR activity (510 mV of the overpotential to reach 10 mA cm −2 ), excellent selectivity (the peak FE of 87 % at 3.34 V vs. RHE), and stability (only 3 % of the FE degradation after 3 h). DFT calculations Density functional theory (DFT) calculations were performed using the Vienna ab initio Simulation Package (VASP) code [69] . The projector augmented wave (PAW) method was used to describe the interactions between electrons and ion cores [70] . The electron exchange and correlation energy were described using the revised Perdew-Burke-Ernzerhof (RPBE) functional [71] . A plane-wave cutoff energy of 500 eV was utilized to expand the wavefunctions. The total energy convergence was set to be lower than 10 −6 eV, and the convergence criterion for geometry optimizations was set to a maximum force of 0.02 eV/Å. U values of 7.0 and 4.5 eV were set for LaNiO 3 and LaCuO 3 , respectively, to describe the strong correlation effect of Ni 3d and Cu 3d by the DFT + U method. Periodic boundary conditions were used in all directions, and the facets of (100), (110), and (111) for LaAlO 3 were investigated. A Monkhorst-Pack grid with dimensions of 4 × 4 × 1 was used for sampling the first Brillouin zones [72] , and 15 Å of vacuum in the z-direction was employed to separate the slabs. The two-electron reaction pathway for WOR can be written as: 
    H_2O+∗→*OH+(H^++e^-)
 
    H_2O+∗→*OH+(H^++e^-)
 
    ∗OH+∗OH→H_2O_2
 The reaction energy of each elementary step for the WOR has been calculated based on the method developed by Nørskov et al. [73] as follows: 
    G= E+ ZPE-T S+G_U+G_pH+G_field
 (1) 
    G_U=eU
 (2) 
    G_pH=0.0592× pH
 (3) where ∆E is the total energy change obtained from DFT calculations, ∆ZPE is the change of zero-point energy, T is the temperature (298.15 K), and ∆S represents the entropy change. 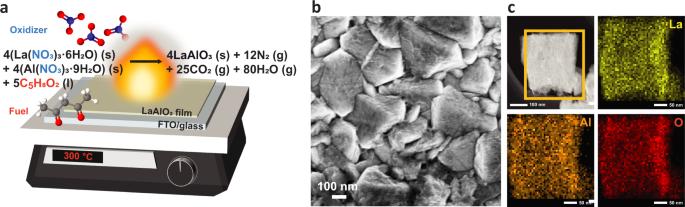U is the electrode potential (vs. reversible hydrogen electrode), and e - is the charge transferred. ΔG field is the free energy correction due to the electrochemical double layer and is neglected as suggested in previous studies [73] , [74] . Fig. 3: Solution combustion synthesis process and characterizations of the final product. aSchematic of low-temperature solution combustion processing mechanism for LaAlO3synthesis.bSEM top-view andcTEM dark-field and EDS mapping images of the synthesized LaAlO3. Zero-point energy and entropies of the adsorbed species were calculated from the vibrational frequencies (Supplementary Table 3 ). We used the computational hydrogen electrode model, which exploits G(H + + e - ) = \(\frac{1}{2}\) G(H 2 ) under pH = 0 and U = 0 V. The free energy of H 2 O was calculated from gas-phase H 2 O at 0.035 bar, 298.15 K. To study the stabilities of (100), (110), and (111) facets for LaAlO 3, we calculated their surface energies using the following equation: 
    =(E_tot-N_La∗E_bulk)/N
 (4) where E tot and E bulk . refer to the total energies of the structures with a specific facet and unit bulk, N La and \({{\mbox{N}}}\) refers to the numbers of Lanthanum and total atoms, respectively. Computational screening A large library of more than 2000 perovskites has been investigated using high-throughput screening. In the first step, we set the stability criteria to E above hull ≤ 0.1 eV to filter the stable perovskites. Next, we used the Pourbaix diagram to predict the compositions of oxides and identify the electrochemical stability of perovskites under different reaction conditions (various pH and potentials). Pourbaix diagram was constructed by using Python Material Genome (Pymatgen) [48] and Materials Project [40] . Sample preparation All chemical precursors were purchased from Sigma Aldrich. We deployed the acetylacetone-based sol-gel combustion synthesis. First, 0.2 M of La(NO 3 ) 3 ·6H 2 O and Al(NO 3 ) 3 ·9H 2 O were dissolved in 5 ml of 2-methoxyethanol in a 1:1 ratio, followed by 0.2 ml of acetylacetone. After completely dissolving the metal salts, 114 µl of NH 4 OH was added to the solution. Then, the solution was aged for 12 h. Next, the 80 µl of the precursor solution was spin-coated on the cleaned fluorine-doped tin oxide (FTO, 7–8 ohm/sq, MSE supplies) substrate at 3000 rpm for 20 s, then annealed at 300 °C for 30 min under air. Here, a combustion-based synthetic approach is applied to oxide thin films, using acetylacetone as a ‘fuel’ and metal nitrates as oxidizers [58] . Materials characterizations Sample morphology was investigated using scanning electron microscopy (SEM, FEI Magellan 400), and high-resolution, dark-field, and energy-dispersive X-ray spectroscopy (EDS) mapping images were collected by transmission electron microscopy (TEM, FEI Tecnai G2 F20 X-TWIN, 200 kV) at Stanford Nano Shared Facilities (SNSF). The TEM instrument was run using the TIA interface, and Gatan Digital Micrograph was employed to calculate the material d-spacing value with a Fast Fourier Transform (FFT) image. Here, d-spacing was determined by the gap between two symmetrical diffraction points in the FFT image. Grazing-incidence X-ray diffraction (GIXRD) was measured at Beamline 2-1 of the Stanford Synchrotron Radiation Lightsource at SLAC National Accelerator Laboratory with an incident energy of 17.0 keV (0.729 Å) and a Huber 2-circle goniometer. The beam was sliced down to a vertical height of ~ 30 μm and a nominal width of 1 mm. The scattered X-rays were determined using a Pilatus 100 K area detector from Dectris with 487 × 195 pixels (172 μm × 172 μm pixel size). During measurements, the incident angle of the X-ray remained fixed while the detector was moved through a range of diffraction angles. The surface analysis with an elemental quantification was investigated using X-ray photoelectron spectroscopy (XPS, PHI VersaProbe 3) that uses a monochromatized Al Kα radiation (1486 eV). All XPS spectra were calibrated to the C 1 s peak at a binding energy of 284.8 eV. CasaXPS software was used to carry out peak fitting with Shirley backgrounds. Thermogravimetric and differential scanning calorimetry (TGA/DSC, Setaram Labsys Evo) were simultaneously used to obtain the heat flow and mass change on the precursor solution with the temperature range from 25 to 800 °C at a heating rate of 10 °C/min. Electrochemical measurement Electrochemical measurement was conducted using a potentiostat (Model Interface 1010, Gamry) and three-electrode electrochemical cell including LaAlO 3 /FTO working electrode (geometric area of 0.502 cm 2 ), carbon rod counter electrode [75] , [76] , and Ag/AgCl (KCl Sat.) reference electrode in the 30 mL of the electrolyte of 2 M KHCO 3 (pH 8.3) and 4 M K 2 CO 3 /KHCO 3 (1:7, pH 11). The measured potentials versus Ag/AgCl were converted to the potentials versus reversible hydrogen electrode (RHE) by the equation below: 
    E_RHE=E_Ag/AgCl+0.059×pH+0.197
 (5) The electrochemical activity was evaluated using linear sweep voltammetry (LSV), sweeping from 1.2 V to 2.4 V vs. RHE at a scan rate of 50 mV/s. All curves are 95% iR-compensated. The EIS measurement was conducted between 20 kHz and 0.05 kHz at 2.7 V vs. RHE for all samples. Chronoamperometry assessed stability, applying a constant potential of 2.7 and 3.2 V vs. RHE for 3 h. H 2 O 2 was collected during the chronoamperometry test at different times, followed by UV-vis absorbance measurement of the mixture solution of cobalt sulfate and the electrolyte, including the produced hydrogen peroxide. Before measuring the absorbance, the complexation time is required for 30 min. A calibration curve was measured with the same procedure but using commercial hydrogen peroxide [9]. H 2 O 2 with higher concentration was quantified using the titration method with potassium permanganate and sulfuric acid, based on the following reaction: 
    2MnO_4^-(aq) +6H^+(aq) + 5H_2O_2(aq) → 2Mn^2+(aq) +8H_2O (l) +5O_2(g)
 Selectivity was evaluated by the calculation of Faradaic efficiency, which is determined by the equation below: 
    FE=n×N_H_2O_2× F/I× t
 (6) where n, N H2O2 , F, I, and t represent the number of electrons, the mole of H 2 O 2 produced, faradaic constant, measured current, and time, respectively. The FEs at each potential were calculated by applying the absorbance measurement from its calibration curve (Supplementary Fig. 23 ) after the chronoamperometry test for 10 min, as shown in the Methods section. The inset picture in Supplementary Fig. 23 indicates the mixture of cobalt sulfate dye and the electrolyte, including the generated H 2 O 2 : the more greenish the solution looks, the more H 2 O 2 is generated.